A guideline for atomistic design and understanding of ultrahard nanomagnets Magnetic nanoparticles are of immense current interest because of their possible use in biomedical and technological applications. Here we demonstrate that the large magnetic anisotropy of FePt nanoparticles can be significantly modified by surface design. We employ X-ray absorption spectroscopy offering an element-specific approach to magnetocrystalline anisotropy and the orbital magnetism. Experimental results on oxide-free FePt nanoparticles embedded in Al are compared with large-scale density functional theory calculations of the geometric- and spin-resolved electronic structure, which only recently have become possible on world-leading supercomputer architectures. The combination of both approaches yields a more detailed understanding that may open new ways for a microscopic design of magnetic nanoparticles and allows us to present three rules to achieve desired magnetic properties. In addition, concrete suggestions of capping materials for FePt nanoparticles are given for tailoring both magnetocrystalline anisotropy and magnetic moments. The small size of magnetic nanoparticles opens new fields of applications from the technological and biomedical perspective [1] , [2] . They can be used, for example, as new ultrahigh density magnetic storage media or as contrast agents in magnetic resonance imaging techniques, as controllable drug carrier, and as material for hyperthermia treatment. These innovative applications based on ultrasmall magnetic objects in biomedical theranostics, water treatment and multifunctional materials require an atomistic understanding and control of magnetic properties like the orientation and magnitude of the atomic magnetic moment. Current efforts further concentrate on improving permanent hard magnets, which are required for future energy-harvesting technologies [3] , while recently also exchange-spring composites based on soft and hard magnetic nanoparticles have been discussed for advanced applications of permanent magnets [4] . Another example is the combination of catalytic activity with magnetic response [5] . Designing new types of bimetallic multifunctional nanoparticles for all of these applications requires the atomistic understanding of the origin of the particles' magnetism, for example, if it is dominated by the large surface fraction of the atoms in a lower coordinated electronic state or dominated by intrinsic lattice strains. For instance, the use of FePt nanoparticles as magnetic storage media, with the magnetization direction of one single particle representing one bit, has been discussed for more than a decade. A significant increase of the storage density requires a drastic decrease of the nanoparticle size. However, the small size of nanostructures is boon and bane. In nanoparticles, thermal fluctuations may lead to a decay of the stable magnetization direction, termed as 'superparamagnetism', which inhibits long-term data storage. The coupling of the magnetization direction to the crystal lattice of the material by spin-orbit and magnetic dipole interaction is usually described by the effective magnetic anisotropy energy (MAE) density K eff . The larger K eff , the smaller the critical particle size for stable magnetization at room temperature. As FePt in the chemically ordered L1 0 state is one of the materials with the highest value of the effective MAE density, K eff =6×10 6 J m −3 (refs 6 , 7 , 8 ), it has been considered as the prime candidate for future data storage media application. Using this value for FePt nanoparticles and assuming a minimal stability ratio of stored magnetic information ( K eff V ) to the thermal energy ( k B T ), K eff V /( k B T )≈50–70, stable grains down to sizes of about d ≈(60 k B T / K eff ) 1/3 ≈2.5 nm are conceivable [9] . However, for nanoparticles of FePt alloys, K eff is reduced by about one order of magnitude [10] , [11] , but still large compared with other ferromagnetic materials like, for example, bcc Fe. One also has to consider that the MAE is strongly influenced by lattice parameters and symmetry decreasing distortions [12] . In particles, these can be altered with respect to the bulk case by interlayer relaxation [13] due to the presence of facetted surfaces or surface tension. For technological applications, particles need to be deposited on surfaces or embedded in a host material, which may cause structural deformations leading to an unknown modification of the desired properties. Also, the particles may have to be exposed to a more or less reactive atmosphere from which they can be protected by deliberately covering them with suitable elements. The presence of a different chemical surrounding, however, provides an electronic environment of the surface (interface) atoms with a tendency to alter the hybridization of the d states, which are responsible for the large MAE. In nanoparticles with a nearly balanced surface-to-volume ratio, both effects on the MAE, structural and electronic, will be significant. It is the purpose of this work to quantify these contributions in atomistic detail by means of a combined experimental and theoretical investigation. We present the results on the influence of surface modifications on the MAE and the magnetic moments by capping FePt nanoparticles with Al, Au or Cu studied by large-scale first-principles calculations within the framework of density functional theory (DFT) and X-ray absorption spectroscopy and its associated magnetic circular dichroism (XMCD). This combined effort provides the unique possibility to simultaneously determine the MAE and microscopic magnetic properties like the spin and orbital magnetic moments. While the spectroscopic investigations rather provide averaged values per atom deduced from nanoparticle ensembles, the DFT ideally complements the experiment by allowing the quantitative calculations of structural and electronic properties on the atomistic level for individual particles. The link to the electronic structure helps to understand the relevant properties and to design guidelines for improved materials. Orbital magnetism of ultrathin films or nanostructures has been a topic of intense theoretical research for more than two decades [14] , [15] , [16] , [17] . Up to now, the main efforts have gone into understanding the intriguing properties of ultrathin magnetic layers on non-magnetic substrates [18] , [19] , while the inverse problem, the influence of non-magnetic layers on magnetic substrates, has attracted much less attention. The presence of several non-equivalent surfaces and the possibility of surface-related relaxation effects affecting the particle core, however, call for a new integral approach, paying attention to the influence of all relevant interfaces at the same time. The merit of such an approach is demonstrated in the present investigation. Furthermore, our atomistic approach allows the evaluation and prediction of artificial structures that do not exist in nature. We will demonstrate below that this can be used to separate hybridization effects with capping materials from the influence of intrinsic distortions of the particle itself. Orbital and spin magnetic moments Site-specific magnetic moments were calculated within DFT for chemically ordered Fe 67 Pt 80 and Fe 80 Pt 67 cuboctahedra in the L1 0 structure covered by an additional layer of Al, Cu or Au. After geometrical relaxation by minimization of the total energy, it can be clearly seen that the morphology of the FePt nanoparticle is almost unaffected by Cu and Au layers, while Al coverage causes severe changes of shape and crystal structure ( Fig. 1 ). The spin-orbit contribution of an electron to the Hamiltonian is generally expressed by the relation H SOC = ξ l·σ , where σ and l refer to spin and orbital momenta, respectively, and ξ is the spin-orbit-coupling parameter. The latter is about one order of magnitude larger for the 5d elements like Pt, while the opposite holds for the exchange splitting of the 3d component Fe. Thus, for FePt none of the elemental contributions may be neglected a priori . A detailed inspection of the individual spin and orbital moments of the FePt core, as presented in Figure 2 , will therefore be necessary to identify the relevant trends. 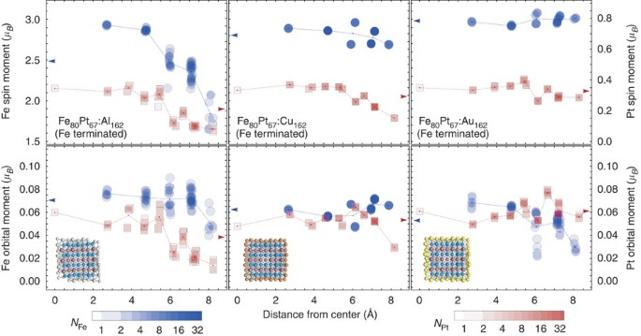Figure 2: Calculated orbital and spin magnetic moments of Fe and Pt atoms in capped FePt nanoparticles. Spatially resolved spin (top) and orbital (bottom) moments of the Fe and Pt atoms for Al-, Cu- and Au-covered Fe80Pt67nanoparticles, with (001) surfaces of Fe. The moments are shown as a function of their distance from the particle centre. Blue circles denote position and moments of Fe atoms, while reddish squares depict Pt. The intensity of the colour refers on a logarithmic scale to the number of overlapping symbols, that is, the frequency of atoms with a given moment and distance from centre. The dashed lines connect the averages of distances and moments over all atoms of the respective species, which belong to the same fcc coordination shell; the arrow heads at the left and right axis denote the respective nanoparticle averages of Fe and Pt moments. 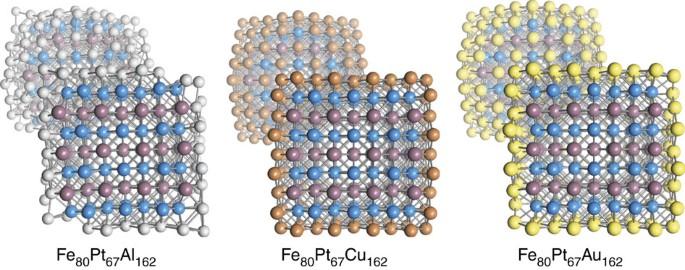As the particle shape is close to spherical, the quantities are presented site-resolved with respect to their distance to the particle centre. Figure 1: Morphology of capped FePt nanoparticles. L10Fe80Pt67nanoparticles terminated with a monolayer of Al, Cu and Au after structural relaxation. Blue spheres refer to Fe, reddish spheres to Pt atoms and the other colours to the respective covering element. The foreground shows the nanoparticles in cross-section. Figure 1: Morphology of capped FePt nanoparticles. L1 0 Fe 80 Pt 67 nanoparticles terminated with a monolayer of Al, Cu and Au after structural relaxation. Blue spheres refer to Fe, reddish spheres to Pt atoms and the other colours to the respective covering element. The foreground shows the nanoparticles in cross-section. Full size image Figure 2: Calculated orbital and spin magnetic moments of Fe and Pt atoms in capped FePt nanoparticles. Spatially resolved spin (top) and orbital (bottom) moments of the Fe and Pt atoms for Al-, Cu- and Au-covered Fe 80 Pt 67 nanoparticles, with (001) surfaces of Fe. The moments are shown as a function of their distance from the particle centre. Blue circles denote position and moments of Fe atoms, while reddish squares depict Pt. The intensity of the colour refers on a logarithmic scale to the number of overlapping symbols, that is, the frequency of atoms with a given moment and distance from centre. The dashed lines connect the averages of distances and moments over all atoms of the respective species, which belong to the same fcc coordination shell; the arrow heads at the left and right axis denote the respective nanoparticle averages of Fe and Pt moments. Full size image The presence of an Al cap leads to a significant reduction of the Fe spin polarization in the interface region, which induces a simultaneous breakdown of the Pt spin and orbital moments. This strong effect of the hybridization of the Fe 3d states with additional (s, p) electrons suggests that elements of the Au group may be a better alternative to minimize the impact of the matrix on the magnetic properties of the particle, while reducing the tendency of interdiffusion of particle and matrix elements. Indeed, our calculations concerning Cu-covered particles reveal no impact on the magnetism of the Fe atoms, only a moderate reduction of the Pt spin magnetic moment. In the case of Au capping, solely the Fe orbital moment is affected. This suggests that in the first case the Pt-terminated while in the second case the Fe-terminated surface should rather be avoided, respectively, in order to get magnetic moments close to the values of uncapped FePt nanoparticles. This clearly shows that not only the choice of the appropriate covering element is important, but also the termination at the particle interface can have a major impact on spin-orbit-related properties, which consequently should be accounted for during the fabrication process of the particle itself. For all ternary systems, we find that the characteristic site-dependent variation of the Pt spin moments is accompanied by a likewise pattern shown by the respective orbital moments. This demonstrates that in accordance with previous considerations for the bulk case [20] , [21] , the orbital magnetism of Pt is dominated by single-site contributions due to the large spin-orbit-coupling parameter, even close to the interface. This leads to the primary guideline that preserving a large Pt spin magnetic moment at the interface is crucial for maintaining the desired hard magnetic properties. A similar correspondence is not encountered for the 3d species, which is affected via hybridization by the strong spin-orbit coupling to the 5d sites [22] . In order to prove the calculated results experimentally, we focus on the determination of element-specific magnetic moments and MAE of FePt nanoparticles with different sizes (6 and 2 nm) capped with Al. These should show the strongest modification on structure and magnetism compared with the uncapped case. Light elements like Al and its passivating surface oxides do not impose technical problems in measuring the X-ray absorption near-edge structure (XANES) by total electron yield as discussed in the Supplementary Information . 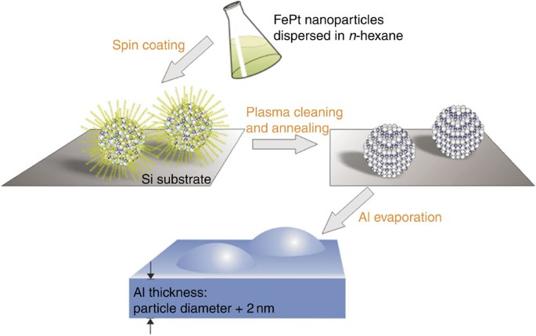Figure 3: Preparation steps. Schematic overview of sample preparation of pure metallic, that is, oxygen-free and ligand-free, FePt nanoparticles capped with Al. The wet-chemically synthesized FePt nanoparticles [23] were deposited onto a naturally oxidized Si substrate as depicted in Figure 3 . 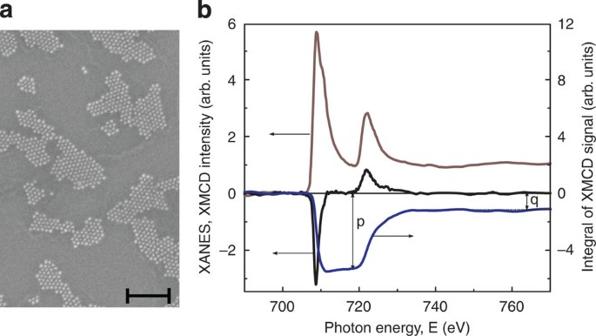Figure 4: Experimental X-ray absorption data of an FePt nanoparticle ensemble capped with Al. (a) Exemplary scanning electron microscopy image of uncapped 6 nm FePt nanoparticles on a naturally oxidized Si wafer. (b) X-ray absorption near edge structure (reddish line) and its associated magnetic circular dichroism (black line) at the Fe L3,2absorption edges. Integrating the dichroic spectrum (blue line) yields the element-specific magnetic moments at the Fe sites. A typical scanning electron microscopy image is shown in Figure 4a . By an oxygen and subsequent hydrogen plasma treatment [24] , all organic ligands (oleic acid and oleylamine) surrounding the particles in the as-prepared state are removed completely and oxides are reduced. After this cleaning procedure, the particles were annealed in order to obtain the chemically ordered L1 0 state and capped with Al. In order to avoid interface alloying, the sample was allowed to reach room temperature again after annealing and before evaporation of Al was started. However, some interdiffusion at the interface cannot be excluded entirely. More details on the sample preparation can be found in the Supplementary Information . The thickness of the Al was chosen to be 2 nm larger than the mean diameter of FePt nanoparticles to prevent the particles from oxidation, that is, 4 nm for the particles with 2 nm in diameter and 8 nm for the particles with 6 nm in diameter, respectively. As Al forms a passivating oxide layer that is only about 1 nm thick when exposed to air, the thickness of Al capping is sufficient to ensure a pure, that is, non-oxidized FePt/Al interface. Figure 3: Preparation steps. Schematic overview of sample preparation of pure metallic, that is, oxygen-free and ligand-free, FePt nanoparticles capped with Al. Full size image Figure 4: Experimental X-ray absorption data of an FePt nanoparticle ensemble capped with Al. ( a ) Exemplary scanning electron microscopy image of uncapped 6 nm FePt nanoparticles on a naturally oxidized Si wafer. ( b ) X-ray absorption near edge structure (reddish line) and its associated magnetic circular dichroism (black line) at the Fe L 3,2 absorption edges. Integrating the dichroic spectrum (blue line) yields the element-specific magnetic moments at the Fe sites. Full size image An example of XANES and XMCD measured at the Fe L 3,2 absorption edges of an ensemble of pure metallic 6 nm FePt nanoparticles covered with Al is shown in Figure 4b . A small shoulder that is visible above the L 3 absorption edge around 710 eV could be assigned to a hybridization between Fe d-states and Al sp-states as it is known, for example, for the similar case of Fe d-states and Si sp-states in Fe 3 Si [25] . Evidence for this can be found in the electronic density of states. This hybridization yields also a reduction of the XMCD in the energy range between 710 and 715 eV compared with Fe bulk material, which is also useful to distinguish between the changes in the spectral shape of the XANES caused by hybridization with Al states and the formation of Fe oxides that show a different XMCD signal (see for example, ref. 26 ). By integration of the XMCD, the total magnetic moment per unoccupied final states at the Fe sites can be separated into spin and orbital contribution according to the so-called sum rules [27] , [28] , [29] . The values are listed in Table 1 using a number of unoccupied d-states n h =3.41 obtained from band structure calculations. Note that the values taken from ref. 30 have been recalculated with the same number of unoccupied d-states. As predicted by theory, the magnetic moments at the Fe sites of Al-capped FePt particles with diameters around 6 nm are significantly reduced with respect to the ones of uncapped nanoparticles of the same size [30] . Increasing the fraction of surface atoms by reducing the particle diameter yields a further decrease of spin and orbital magnetic moments indicating that the magnetic moments of Fe atoms at the interface to the Al cap layer are significantly reduced as it was already expected from our theoretical investigations. The total magnetization can be estimated by summing up the experimentally determined spin and orbital magnetic moments per unit cell volume, V ≈(0.386 nm) 3 . For uncapped particles, both Fe and Pt magnetic moments were determined as reported elsewhere [31] yielding a magnetization M ≈10 6 A m −1 . For Al-capped particles, the Pt moments are assumed to be reduced with respect to the ones measured for uncapped FePt nanoparticles by the same factor as the Fe magnetic moments, that is, about 10% for 6 nm particles yielding a total magnetization M ≈9×10 5 A m −1 , and about 25% for 2 nm particles yielding M ≈7.5×10 5 A m −1 , respectively. Table 1 Fe XMCD results * . Full size table Note that the ratio of orbital-to-spin magnetic moment remains unchanged within experimental error. Compared with our theoretical results, this may indicate a Fe-terminated surface of the wet-chemically synthesized nanoparticles. Magnetic anisotropy The proportionality between the anisotropy of orbital magnetic moments and MAE proposed by Bruno [14] for elementary metals was put into question for binary 3d–5d systems [22] , [31] . Consequently, for FePt it is necessary to determine the MAE independently, for example, by recording the field-dependent XMCD as a measure of magnetization [32] at various temperatures. 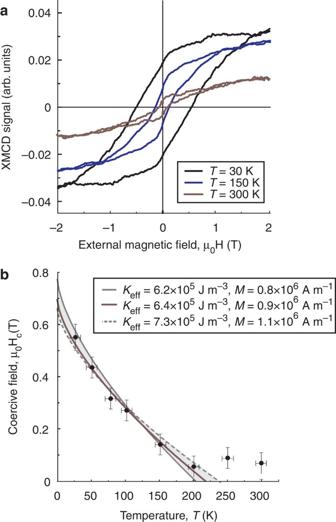Figure 5: Field- and temperature-dependent XMCD measurements for the estimation of magnetocrystalline anisotropy. (a) Field-dependent X-ray magnetic circular dichroism as a measure of magnetization at the Fe sites of Al capped FePt nanoparticles for three different temperatures. (b) Extracted temperature dependence of the coercive field (filled symbols) and simulations using Sharrock's equation with different parameters (lines). Note that for FePt, 1×106J m−3corresponds to ~0.1 meV per atom (0.2 meV per Fe atom, respectively). Examples at three different temperatures can be seen in Figure 5a . For ensembles of non-interacting nanoparticles with diameter d, uniaxial anisotropy K eff and randomly oriented easy axes of magnetization, the temperature dependence of coercivity can be described by Sharrock's equation [33] : Figure 5: Field- and temperature-dependent XMCD measurements for the estimation of magnetocrystalline anisotropy. ( a ) Field-dependent X-ray magnetic circular dichroism as a measure of magnetization at the Fe sites of Al capped FePt nanoparticles for three different temperatures. ( b ) Extracted temperature dependence of the coercive field (filled symbols) and simulations using Sharrock's equation with different parameters (lines). Note that for FePt, 1×10 6 J m −3 corresponds to ~0.1 meV per atom (0.2 meV per Fe atom, respectively). Full size image Simulation of the experimental data as shown in Figure 5b yields an effective anisotropy of K eff =6–7×10 5 J m −3 corresponding to a mean blocking temperature of about 220 K. This approximately agrees with earlier experiments on uncapped nanoparticles [10] , [34] . For the simulations, the magnetization was varied around the value estimated from the magnetic moments as described above. The non-vanishing coercivity above the mean blocking temperature is related to nanoparticles with larger diameters than the mean value of 6 nm. From theory, the influence of capping layers on the MAE can be determined by the differences in the band energies obtained by changing the magnetization direction away from the easy axis parallel to the shortened c axis of the L1 0 lattice to the (intermediate) hard axis perpendicular to it. The results for the different possibilities of surface termination ( Fig. 6 ) indicate in fact a large influence of the capping species, and corroborate the trends obtained from the orbital moments above. While Al capping leads to a significant decrease of the MAE regardless of the termination of the FePt (001) facets, the elements with the filled d shell, Cu and Au, yield encouraging results coming close to the values obtained for uncapped nanoparticles. Cu and Au are iso-electronic, they only differ by size and the location of the centre of the d-band with respect to the Fermi energy as well as magnitude of the spin-orbit-coupling parameter. Computer experiments offer full control of the configurational arrangements and thus provide a straightforward possibility to estimate the contribution from matrix-induced geometrical changes, which will, for example, arise from a variation of the tetragonal distortion of the particle core [35] . We can estimate such contributions by removing all covering atoms but leaving the Fe and Pt atoms exactly in place. The MAE of the stripped nanoparticles is for all cases significantly larger than the MAE of the original decorated isomers, which can be naturally traced back to the released quenching of orbital magnetism of the surface atoms. The MAE of the stripped nanoparticles can significantly exceed the values obtained for the fully relaxed isomers with clean surfaces, whereas the electronic interaction with the atoms of the capping layer generally leads to a reduction of the MAE. These results demonstrate clearly that both structural modifications due to additional layers of surface atoms and changes in the electronic environment, yield equally important contributions, which need to be taken into account explicitly when comparing experimental results on free nanoparticles, embedded nanoparticles and nanoparticles supported by different substrates. 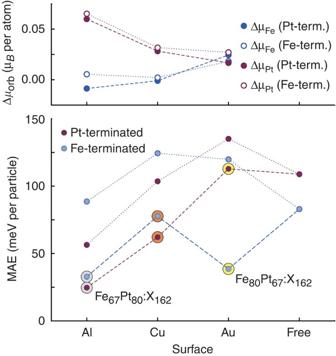Figure 6: Calculated magnetocrystalline anisotropies for capped FePt nanoparticles. Comparison of the calculated magnetocrystalline anisotropy energy (MAE) in meV per atom for different cappings and termination of the (001) surfaces. The small circles refer to 147 atom particles with stripped decorations but retained atomic positions and clean nanoparticles. The values have been calculated relying on the magnetic force theorem from the difference in band energy between the easy and intermediate axis orientations of collinear magnetic arrangements in [001] and [100] directions. The upper panel shows the difference Δμorb=μstripped−μdecoratedbetween the average orbital moment between stripped and decorated configurations (magnetization ║ [001]). Note that a value of 100 meV per particle corresponds to ~7×106J m−3. Figure 6: Calculated magnetocrystalline anisotropies for capped FePt nanoparticles. Comparison of the calculated magnetocrystalline anisotropy energy (MAE) in meV per atom for different cappings and termination of the (001) surfaces. The small circles refer to 147 atom particles with stripped decorations but retained atomic positions and clean nanoparticles. The values have been calculated relying on the magnetic force theorem from the difference in band energy between the easy and intermediate axis orientations of collinear magnetic arrangements in [001] and [100] directions. The upper panel shows the difference Δ μ orb = μ stripped − μ decorated between the average orbital moment between stripped and decorated configurations (magnetization ║ [001]). Note that a value of 100 meV per particle corresponds to ~7×10 6 J m −3 . Full size image In the case of Au coverage, the change of the interface termination from Fe to Pt is connected with a strong increase of the MAE, which—following ref. 33 —can be related to contributions from off-site spin-orbit scattering of the Fe states, which seem also to be responsible for the quenching of the interfacial orbital magnetic moments of Fe as shown in the upper panel of Figure 2 . Thus, the type of the particle's surface termination can be deemed of particular importance if the protective shell consists of heavy elements, which possess a large spin-orbit-coupling parameter. Note that also other coverages have been considered in our calculations, such as carbon, as presented in the Supplementary Information . In that case, the hybridization of the (s, p) states of C with the d states of FePt is presumably strong, and the magnetism of the FePt nanoparticle further suffers from the diffusion of C into the FePt particle matrix. We expect that this negative aspect of C capping will survive for other covalently bonding materials as well. Our combined approach allows us to disentangle the different contributions that strain and surface modifications have on the magnetic properties of free and covered magnetic nanoparticles by correlating detailed experimental and ab initio large-scale DFT calculations. From our results, we will deduce basic fabrication guidelines to appropriately modify the magnetic properties, that is, MAE and magnetic moments, by capping FePt nanoparticles in L1 0 symmetry: in order to obtain protected hard magnetic nanostructures with large MAE, one must ensure in the first place that the spin moment of the Pt interface atoms will not be affected by the capping—neither directly, nor indirectly by quenching of the inducing Fe moments, unless the presence of a soft magnetic shell (or possibly even a dead layer) is desired. Exactly this is the case if the protective cover allows for hybridization with (s, p) electrons. Unaffected by experimental difficulties in the XANES measurements, the DFT approach straightforwardly allows us to inspect site-resolved orbital magnetism of particles capped with heavier elements, as the late elements of the d series. Indeed, Cu and Au present alternatives preserving the hard magnetic properties of the FePt core. In the case of Au, however, additional attention must be paid to the specific interface contributions to the MAE according to the interaction with the different facets of the magnetic core. Decoration of carefully selected facets with sixth row elements can thus provide a significant improvement over a mere minimization of anisotropy losses. The corresponding interactions are, however, not easily predictable a priori , and the magnetic properties of such nanocompounds can decisively depend on the fabrication conditions. An interesting option for a further systematic investigation may also be capping with elements of the 5f series as their degree of electron localization increases with the atomic number from itinerant (taking part in the chemical bond) to strongly localized (comparable, for example, with rare earth metals) while large orbital magnetic moments are present. Our findings can be condensed into three key observations, which form the basic ingredients to construct guidelines for the design of FePt nanoparticles with special magnetic properties. First, as not only the choice of the appropriate covering element is important, but also the termination at the particle interface can have major impact on the MAE, it is necessary to select the appropriate surface termination within the fabrication process. Second, preserving a large spin magnetic moment at the Pt sites at the interface is crucial for maintaining the hard magnetic properties of FePt (as the hybridization of the 5d states with the strongly spin polarized 3d states of Fe is essential for a large magnetocrystalline anisotropy). Third, structural modifications due to additional layers of surface atoms and changes in the electronic environment are equally important for the magnetic properties. These observations imply that it is possible to design nanoparticular systems with the desired magnetic properties by choosing the right capping material from a technological perspective or for basic research. The origin of these different magnetic properties for different capping materials is due to both electronic hybridization effects and structural distortions of the nanoparticle itself, which can be separated by means of state-of-the art first-principles calculations. Consequently, our combined approach allows us to formulate three design rules for L1 0 FePt nanoparticles with optimized magnetic properties. First, for hard magnetic FePt nanoparticles: to maintain the large MAE of uncapped FePt nanoparticles and their magnetic moments, covering with an element from the late d series like Cu is advised. For FePt nanoparticles with Pt-terminated surfaces, capping with Au gives the possibility to even exceed the MAE of the uncapped particles. Second, for soft magnetic FePt nanoparticles with large saturation magnetization: FePt nanoparticles with Fe-terminated surfaces should be capped with heavy elements with large spin-orbit coupling like Au, which yield largely unchanged magnetic moments with respect to the uncapped particles, but a significant decrease of the MAE. Third, for soft magnetic FePt nanoparticles with reduced saturation magnetization: capping with Al yields to a significant reduction of both MAE and magnetic moments. Lighter elements like C show enhanced diffusion into the particle and yield to a complete breakdown of the net magnetization. Calculations Structural relaxations were carried out in the framework of DFT and the Vienna Ab-initio Simulation Package [36] . The wavefunctions of the valence electrons (3d 7 4s 1 for Fe, 5d 9 6s 1 for Pt, 3s 2 3p 1 for Al, 3d 10 4s 1 for Cu and 5d 10 6s 1 for Au) were expanded within a plane wave basis set (cutoff E cut =335...450 eV) in combination with the PAW method for the interaction with nuclei and core electrons [37] . We used the generalized gradient approximation exchange correlation functional in the formulation of Perdew and Wang [38] , [39] together with the spin interpolation formula of Vosko, Wilk and Nusair [40] . Spin-orbit interaction can be included in the non-collinear version of the code [41] , [42] , [43] . For each of the core-shell particles (FePt/Al, FePt/Cu and FePt/Au), we considered 147 atom FePt clusters (consisting of 67 Fe atoms and 80 Pt atoms, and vice versa), with perfect L1 0 layering, capped with 162 atoms of Al, Cu or Au. The particles were placed in a cubic supercell with an edge length of 28 Å to avoid interactions between the periodic images. Geometrical optimizations were carried out on the Born–Oppenheimer surface without any symmetry constraints on charge density and forces using a conjugate gradient algorithm, in a similar manner as in previous investigations of the authors (for further details, see, for example, refs 12 , 44 ). As the problem is non-periodic, Brillouin zone sampling was restricted to the Γ-point with a Gaussian-type finite temperature smearing of the occupancies near the Fermi surface. For the calculation of spin-orbit-related properties extremely well-converged wave functions and charge distributions on the one hand, and a sharp definition of the energy levels close to the Fermi surface on the other are mandatory. To ensure this, the finite temperature smearing was reduced in three consecutive scalar-relativistic calculations with collinear spin alignment with respective widths of σ =50, 20 and 10 meV, the latter initialized by the converged charge density and wave functions of the previous run with larger smearing. The resulting wave functions and charge densities have been used to initialize fully self-consistent calculations of spin and orbital moments with magnetization aligned in the easy axis direction ( E cut =335 eV). These calculations were allowing for possible non-collinear arrangements. However, only minor directional deviations of the spin moments from the easy direction were encountered, which are not significant for the present study. The accurate calculation of the magnetocrystalline anisotropy energy (MAE) requires increased numerical efforts compared with the orbital moments. In agreement with the experience of Błoński and Hafner [43] , an increased energy cutoff of E cut =450 eV and in addition a denser Fourier grid has been chosen. Calculations of this kind are extremely demanding with respect to computation time and memory, and can—so far—for large systems of 300 magnetic transition metal atoms (and beyond) only be performed on world-leading supercomputers as the IBM Blue Gene/P installation JUGENE at Forschungszentrum Jülich, which gave us the possibility to distribute one single calculation on 1,024 compute nodes (or more), simultaneously. A fully self-consistent non-collinear calculation for hard magnetic materials as FePt may yield spurious results as the spin moments are allowed to rotate towards their easy axis. To prevent this, our calculations were carried out in terms of the magnetic force theorem [45] , [46] . Here, non-self-consistent calculations of the relativistic energies are performed for different orientations of the spin quantization axis depending on charge densities and wavefunctions obtained from self-consistent collinear scalar-relativistic runs. The MAE is obtained from the difference in band energies between hard and easy axis (in the present case [001] and [100], the MAE with respect to [110] are in agreement within numerical error). The orbital moments obtained from the non-self-consistent calculations with easy axis alignment were found in close agreement with the above-described fully self-consistent approach. In the main manuscript, spatially relsoved spin and orbital moments were only shown for Fe 80 Pt 67 particles with Fe-terminated (001) surfaces. The results for the Pt-terminated Fe 67 Pt 80 particles are completely analogous and shown for completeness in the Supplementary Figure S1 . In addition to the metallic elements Al, Cu and Au, we also considered an alternative coating of the Fe–Pt clusters with carbon. During the relaxations, we encountered very severe structural distortions, which included (energetically downhill) diffusion of carbon atoms into subsurface positions of the comparatively open [100] and [001] surfaces. Furthermore, we also encountered a dramatic disturbance of surface/interface magnetism, including antiferromagnetic admixtures on the Fe sites, and a nearly complete breakdown of the spin polarization of the interface Pt atoms, as shown in the Supplementary Figure S2 . We attribute, as in the case of Al, this degradation of the magnetic properties to the increased hybridization between d and (s, p) electrons due to the presence of carbon. Sample preparation FePt nanoparticles were synthesized by thermal decomposition of Fe(CO) 5 and Pt(acac) 2 as described elsewhere [23] . The particles are in the chemically disordered state as the formation of the chemically ordered state—which is the equilibrium state at room temperature—is kinetically suppressed. The size distribution was determined by analysis of transmission electron microscopy images. The mean diameters and the standard deviation of the log-normal size distributions of the two samples investigated in this work are d =6 nm with σ =0.15, and d =2 nm with σ =0.17, respectively. In the as-prepared state, the particles are surrounded by organic ligands, oleic acid and oleyl amine. This prevents agglomeration of the particles while deposited onto a naturally oxidized Si substrate using the spin-coating technique. In order to remove the organic ligands, the sample was cleaned by a radio frequency (13.6 MHz) oxygen plasma treatment for 15 min with a power of 30 W at an oxygen pressure of 5 Pa (0.05 mbar). The oxidized Fe was reduced subsequently by a hydrogen plasma treatment for 40 min with a power of 30 W at a pressure of 8 Pa (0.08 mbar). Note that during the oxygen plasma treatment, a small amount of Cu from the Cu electrode may be sputtered and deposited onto the sample. In order to avoid agglomeration of the particles during thermal treatment, the annealing was performed at quite low temperatures of 575 °C at maximum. The annealing procedure under UHV conditions is the following: heating up the sample from room temperature to 575 °C in 2 h and hold the maximum temperature of 575 °C for 7 h, cool down to 475 °C in 30 min and hold 475 °C for 1 h, cool down to 410 °C in 30 min and hold 410 °C for 1 h, cool down to 360 °C in 30 min and hold 360 °C for 1 h, switch off heating. After annealing, the sample was allowed to reach room temperature again before evaporation of Al was started at rates of 0.1–0.2 nm min −1 to avoid alloying. X-ray absorption experiments X-ray absorption measurements were carried out at the PM3 bending magnet beamline of the BESSYII synchrotron radiation source in magnetic fields up to μ 0 H =±2.8T in total electron yield mode by detecting the sample drain current. XMCD was measured by reversing the direction of magnetic field or helicity of X-rays after each scan varying the energy from 680 to 790 eV. Magnetic hystereses were recorded by detection of the field-dependent X-ray absorption signal at the energy of maximum dichroism (708.6 eV) normalized to the field-dependent absorption in the pre-edge region (700 eV). The sample temperature was stabilized at different temperatures between 11 and 300 K. Details on data analysis can be found in the Supplementary Information . How to cite this article: Antoniak C. et al . A guideline for atomistic design and understanding of ultrahard nanomagnets. Nat. Commun. 2:528 doi: 10.1038/ncomms1538 (2011).